X-ray structure and activities of an essentialMononegavirales L-protein domain The L protein of mononegaviruses harbours all catalytic activities for genome replication and transcription. It contains six conserved domains (CR-I to -VI; Fig. 1a). CR-III has been linked to polymerase and polyadenylation activity, CR-V to mRNA capping and CR-VI to cap methylation. However, how these activities are choreographed is poorly understood. Here we present the 2.2-Å X-ray structure and activities of CR-VI+, a portion of human Metapneumovirus L consisting of CR-VI and the poorly conserved region at its C terminus, the +domain. The CR-VI domain has a methyltransferase fold, which besides the typical S -adenosylmethionine-binding site ( SAM P) also contains a novel pocket ( NS P) that can accommodate a nucleoside. CR-VI lacks an obvious cap-binding site, and the SAM P-adjoining site holding the nucleotides undergoing methylation ( SUB P) is unusually narrow because of the overhanging +domain. CR-VI+ sequentially methylates caps at their 2′ O and N 7 positions, and also displays nucleotide triphosphatase activity. The Mononegavirales order groups five families of monopartite, negative-strand RNA viruses many of which are highly pathogenic and/or contagious; the Filoviridae (of which Ebola virus is a representative), the Bornaviridae (Borna disease virus), the Nyamiviridae (midway virus), the Rhabdoviridae (rabies, vesicular stomatitis virus (VSV)) and the Paramyxoviridae (measles virus, human metapneumovirus (hMPV)). These viruses encode a large RNA polymerase ( L ) (usually >2,000 amino acids) that is crucial to viral replication ( Fig. 1a ). It has two distinct roles to replicate the RNA genome and to transcribe viral mRNA. As such it not only polymerizes RNA but also synthesizes fully methylated cap structures [1] . Capping involves the co-transcriptional addition of a guanosine ( G ) to the first nucleotide (N 1 ) of the nascent RNA chain via a 5′-5′ triphosphate bridge, resulting in a G pppN 1 - structure. Typically, this is followed by methylation of nitrogen 7 ( N 7) of G , giving rise to m G pppN 1 -, and of the 2′-oxygen (2′ O ) of the N 1 ribose ( m G pppN 1m -). The cap protects mRNAs against 5′-exonucleases and promotes RNA transport and translation, while 2′ O -methylation prevents detection by cellular-immunity sensors [2] , [3] , [4] . In Rhabdoviridae , CR-V catalyses cap addition by means of an unconventional polyribonucleotydyl-transferase (PRNTase) reaction where a conserved histidine in CR-V forms a covalent phosphoamide bond with the transcript, resulting in a CR-V-pRNA intermediate. The capped transcript is released after ligation of a G pp to the pRNA. This mechanism differs from capping in eukaryotes and most other viruses, in which a guanylyltransferase (GTase) forms a phosphoamide bond with G p, before transferring it to 5′ppRNA [2] . Paramyxoviridae also contain a PRNTase signature motif in their CR-V domains, suggesting they use the same capping strategy as Rhabdoviridae . In addition, however, paramyxovirus and filovirus L proteins contain a KxxxKxxG sequence (K-K-G motif) at their C termini, reminiscent of a signature motif for eukaryotic GTases, where one of the lysines forms the transient phosphoamide bond with G p in the capping reaction [5] . A C-terminal domain of Rinderpest virus L (containing CR-VI and the downstream K-K-G motif) was shown to form such a bond [6] , leaving open the possibility that Paramyxoviridae use GTase activity for capping. 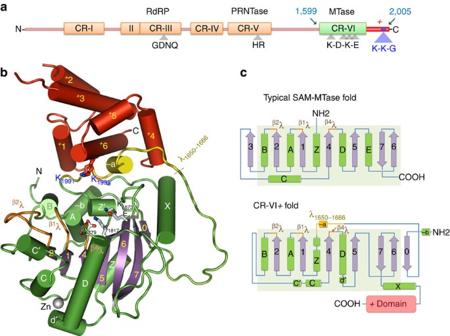Figure 1: The structure of the MTase domain of hMPVL. (a) Domain organization of hMPVL, with at its C terminus the 46.5 kDa CR-VI+ domain (residues 1,599–2,005), comprising CR-VI (green), which contains the K-D-K-E motif typical for 2′O-MTases, and the +domain (red), carrying the K-K-G motif (blue). Boundaries of CR-I to -V are approximate. CR-III contains the G-D-N-Q signature motif for polymerase (RdRP) activity, and CR-V contains the HR motif for PRNTase activity. (b) Cartoon representation of the CR-VI+ crystal structure, from amino (N) to carboxy (C) terminus (no structure could be assigned to the first∼18 residues). The +domain is shown in red, with K1991and K1995of the K-K-G motif in stick format. The CR-VI (MTase) domain is coloured purple (β-strands) and green (helices and loops), except forβ1λ,β2λ andβ4λ (the loop regions C terminal of β-strands 1, 2 and 4 that formSAMP; orange), and λ1650–1666(which disengages itself from the main CR-VI-fold to interact with the +domain; yellow). Nomenclature of helices and strands follows that used for other MTases (c). The pale-blue sticks show the K-D-K-E motif. A Zn-ion (silver sphere) is co-ordinated by H1766, H1798, C1802and C1805. (c) Schematic representation of the secondary structure of a prototypical SAM-dependent MTase (top) and of the hMPV CR-VI domain (bottom). Helices are in green, strands in light purple and coils in blue, except forβ1λ,β2λ andβ4λ (orange) and λ1650–1666(yellow). CR-VI displays some deviations from the prototypical SAM-MTase fold, some of which it shares with other RNA-MTases, including the long N-terminal coil, a longer αD and an extra helix (αX) at the C terminus. αE is absent, whereas, atypical for viral MTases, αB is fully formed. CR-VI, moreover, has an unusual β-sheet; it lacks β3, but this is compensated for by the addition, at the other end of the sheet, of a new strand (β0), which glues the start of the N-terminal coil to the main structure. Also unusual is the fragmentation of αZ (resulting in the small z′-helix). Figure 1: The structure of the MTase domain of hMPV L. ( a ) Domain organization of hMPV L , with at its C terminus the 46.5 kDa CR-VI+ domain (residues 1,599–2,005), comprising CR-VI (green), which contains the K-D-K-E motif typical for 2′ O -MTases, and the +domain (red), carrying the K-K-G motif (blue). Boundaries of CR-I to -V are approximate. CR-III contains the G-D-N-Q signature motif for polymerase (RdRP) activity, and CR-V contains the HR motif for PRNTase activity. ( b ) Cartoon representation of the CR-VI+ crystal structure, from amino (N) to carboxy (C) terminus (no structure could be assigned to the first ∼ 18 residues). The +domain is shown in red, with K 1991 and K 1995 of the K-K-G motif in stick format. The CR-VI (MTase) domain is coloured purple (β-strands) and green (helices and loops), except for β1 λ, β2 λ and β4 λ (the loop regions C terminal of β-strands 1, 2 and 4 that form SAM P; orange), and λ 1650–1666 (which disengages itself from the main CR-VI-fold to interact with the +domain; yellow). Nomenclature of helices and strands follows that used for other MTases ( c ). The pale-blue sticks show the K-D-K-E motif. A Zn-ion (silver sphere) is co-ordinated by H 1766 , H 1798 , C 1802 and C 1805 . ( c ) Schematic representation of the secondary structure of a prototypical SAM-dependent MTase (top) and of the hMPV CR-VI domain (bottom). Helices are in green, strands in light purple and coils in blue, except for β1 λ, β2 λ and β4 λ (orange) and λ 1650–1666 (yellow). CR-VI displays some deviations from the prototypical SAM-MTase fold, some of which it shares with other RNA-MTases, including the long N-terminal coil, a longer αD and an extra helix (αX) at the C terminus. αE is absent, whereas, atypical for viral MTases, αB is fully formed. CR-VI, moreover, has an unusual β-sheet; it lacks β3, but this is compensated for by the addition, at the other end of the sheet, of a new strand (β0), which glues the start of the N-terminal coil to the main structure. Also unusual is the fragmentation of αZ (resulting in the small z′-helix). Full size image Cap methylation is catalysed by S -adenosylmethionine (SAM)-dependent methyltransferases (MTases), which position a SAM molecule next to the target atom on the RNA, enabling the direct transfer of a methyl group and converting SAM into S -adenosylhomocysteine (SAH). In 2′ O -MTases, a conserved K-D-K-E tetrad potentiates methyl transfer [2] . As yet, the boundaries of CR-VI, the putative MTase of L , are not well defined, nor is it clear if CR-VI acts on its own or in conjunction with other domains, whether it mediates both N 7- and 2′ O -methylation and which of these methylations would take place first. Research into the activities of L and the mechanisms underpinning them has historically been hampered by a complete, order-wide absence of high-resolution structures. To redress this, we set out to study L domains of hMPV, a paramyxovirus of the Pneumovirinae subfamily closely related to respiratory syncytial virus (RSV). Like RSV, hMPV is highly contagious and causes respiratory tract disease [7] . As a part of this study, we expressed CR-VI+, a 406-residue fragment comprising CR-VI and the adjoining ‘+ domain’, the variable region carrying the K-K-G-motif, investigated its MTase activity and solved its crystal structure. Besides sequentially methylating the 2′ O and N 7 atoms of small capped RNAs, CR-VI+ also 2′ O methylates uncapped substrates and displays nucleotide triphosphatase (NTPase) activity. Both the CR-VI domain, which assumes a fairly standard MTase fold, and the K-K-G motif of the (mainly helical) +domain are required for the MTase reactions. Combined, the data provide new insights into the modification of the 5′-ends of transcripts emerging from the polymerase domain of L . This structural information on a mononegavirus L protein, and the new insights in the capping mechanism it provides, should spur the development of novel antiviral drugs against this important group of highly pathogenic viruses. MTase activities In vitro , CR-VI+ most effectively binds and methylates synthetic RNAs containing the conserved start sequence of hMPV transcripts, preferring a substrate length of nine nucleotides ( Fig. 2 ). The methylation occurs at the G N 7 and N 1 -2′ O positions ( Figs 2 and 3a ), with 2′ O -methylation preceding N 7-methylation ( Fig. 3a ), an uncommon order of events also occurring in VSV [8] . CR-VI+, moreover, efficiently methylates uncapped RNAs with 5′-phosphate groups (especially pppRNA), primarily at the 2′ O atom of N1 since almost no 3 H-methyl transfer takes place onto the pppG m GGACAAGU substrate where this atom is blocked ( Fig. 2b , green bars). The 2′ O -methylation of pppGGGACAAGU represents ∼ 50% of that observed with G pppGGGACAAGU (which has an extra methylation target in the G N 7 atom; Fig. 2b , red bars). Mutagenesis studies show that all K-D-K-E residues (K 1673 , D 1779 , K 1817 and E 1848 ) are essential for 2′ O -methylation, while the aspartic acid (D 1779 ) in particular is important for N 7-methylation ( Fig. 3b ), as was also observed in Flaviviridae MTases [9] . Other residues, many of which belong to the +domain rather than the core MTase fold, were also found to be essential for the MTase activities (the ‘ SUB P’ residues in Fig. 3b , described below). 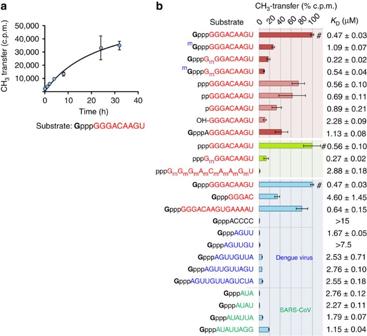Figure 2: MTase activity of CR-VI+. (a). The transfer of tritiated methyl groups from SAM molecules to a capped RNA substrate (GpppGGGACAAGU), containing the consensus start sequence of hMPV transcripts (in red), was monitored over time. The rather slowin vitromethylation suggests the reaction is impaired compared with thein vivoactivity of intactL, regions of which may aid the methyl transfer (for example, by correctly positioning substrate RNAs to the MTase; see main text). The bars and error bars correspond to the mean values from three independent measurements and their s.d.’s, respectively. (b). Substrate specificity was determined as above, but using various synthetic RNA substrates, and allowing the reactions to proceed for 16 h. Substrates were compared withGpppGGGACAAGU (red and blue panels) and pppGGGACAAGU (green panel), for which the degree of methylation was set at 100% (#, marked bars). The red-shaded panel compares the degree of methylation of nine-nucleotide-long hMPV start sequences with different 5′-ends and methylation states (the lighter bars represent uncapped RNAs). The results indicate efficient methylation of RNAs that already carried a (cold) methyl group, either at theirN7-guanine or 2′O-ribose position (confirming the occurrence of 2′O- andN7-methylation, respectively), and of uncapped RNAs (especially pppRNA). The pppRNA substrate is predominantly methylated at N1, as substrates that were methylated beforehand at this nucleotide do not undergo substantial additional methylation (green panel). CR-VI+ prefers the hMPV start sequence over the shortGpppACCCC sequence, and over RNA-start sequences of Dengue virus and SARS coronavirus, irrespective of their lengths (blue panel). A nine-nucleotide hMPV substrate, however, is much preferred over one with only five nucleotides, indicating that additional interactions take place between the protein and nucleotides 6–9. Consistently a 10-times lowerKD(dissociation constant) characterizes the interaction of CR-VI+ with the 9-mer, compared with that with the 5-mer. TheKDs, measured in triplicate using a dot-blot assay and listed at the right of the diagram (±s.d.’s), also show that capped and uncapped hMPV sequences are bound with comparable affinities, and that 2′O-methylated substrates are preferred over unmethylated ones. Figure 2: MTase activity of CR-VI+. ( a ). The transfer of tritiated methyl groups from SAM molecules to a capped RNA substrate ( G pppGGGACAAGU), containing the consensus start sequence of hMPV transcripts (in red), was monitored over time. The rather slow in vitro methylation suggests the reaction is impaired compared with the in vivo activity of intact L , regions of which may aid the methyl transfer (for example, by correctly positioning substrate RNAs to the MTase; see main text). The bars and error bars correspond to the mean values from three independent measurements and their s.d.’s, respectively. ( b ). Substrate specificity was determined as above, but using various synthetic RNA substrates, and allowing the reactions to proceed for 16 h. Substrates were compared with G pppGGGACAAGU (red and blue panels) and pppGGGACAAGU (green panel), for which the degree of methylation was set at 100% (#, marked bars). The red-shaded panel compares the degree of methylation of nine-nucleotide-long hMPV start sequences with different 5′-ends and methylation states (the lighter bars represent uncapped RNAs). The results indicate efficient methylation of RNAs that already carried a (cold) methyl group, either at their N 7-guanine or 2′ O -ribose position (confirming the occurrence of 2′ O - and N7 -methylation, respectively), and of uncapped RNAs (especially pppRNA). The pppRNA substrate is predominantly methylated at N 1 , as substrates that were methylated beforehand at this nucleotide do not undergo substantial additional methylation (green panel). CR-VI+ prefers the hMPV start sequence over the short G pppACCCC sequence, and over RNA-start sequences of Dengue virus and SARS coronavirus, irrespective of their lengths (blue panel). A nine-nucleotide hMPV substrate, however, is much preferred over one with only five nucleotides, indicating that additional interactions take place between the protein and nucleotides 6–9. Consistently a 10-times lower K D (dissociation constant) characterizes the interaction of CR-VI+ with the 9-mer, compared with that with the 5-mer. The K D s, measured in triplicate using a dot-blot assay and listed at the right of the diagram (±s.d.’s), also show that capped and uncapped hMPV sequences are bound with comparable affinities, and that 2′ O -methylated substrates are preferred over unmethylated ones. 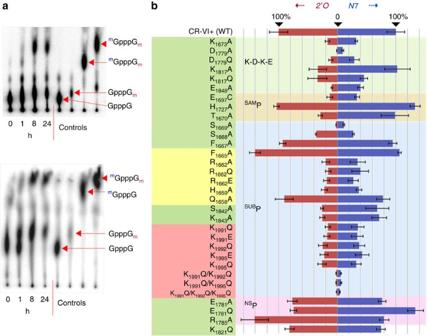Figure 3:N7- and 2′O-methylation. (a) Thin-layer chromatograms. Following CR-VI+-mediated methyl transfer from SAM ontoGpppGGGACAAGU (in whichGwas [32P]-labelled), nucleotides 2–9 were removed by nuclease P1 digestion, and the caps were separated by thin-layer chromatography (TLC). The controls (GpppG,GpppGm,mGpppG andmGpppGm, from left to right) were obtained with the same substrate, using MTases that specifically methylate caps at theN7 or 2′Opositions (humanN7- and vaccinia virus 2′O-MTase). The TLC experiment used 0.65 M LiCl as mobile phase, allowing a clear separation ofmGpppG andmGpppGm(top). The caps on the TLC plate were subsequently further resolved, this time using 0.45 M (NH2)2SO4as mobile phase for a better separation ofGpppG andGpppGm(bottom).GpppGmappears first (after a 1-h incubation),mGpppGmbecomes prominent at a later stage, andmGpppG was not observed, indicating that 2′O-methylation of N1precedesN7-methylation ofG. (b). The effect of point mutations on the MTase activities of CR-VI+, measured after a 16-h incubation period (by means of a filter-binding assay, as inFig. 2), usingGpppGGGACAAGU substrates that were methylated beforehand atN7 ofGor 2′Oof N1, to specifically monitor 2′OorN7-MTase activities, respectively. Mutants are listed against a yellow, green or red background, to indicate that the altered residue belongs to λ1650–1666, the rest of the CR-VI domain, or the +domain, respectively. They are also grouped according to whether they change the K-D-K-E tetrad,SAMP,SUBP orNSP. The results highlight the importance of essentialSUBP residues (such as the K-K-G lysines K1991, K1992and K1995and λ1650–1666residues H1659and R1662) for both 2′O- andN7-methylation. All tetrad residues are crucial for 2′O-methylation, while D1779in particular is important forN7-MTase activity. The bars and error bars correspond to the mean values from three independent measurements and their s.d.’s, respectively. Full size image Figure 3: N 7- and 2′ O -methylation. ( a ) Thin-layer chromatograms. Following CR-VI+-mediated methyl transfer from SAM onto G pppGGGACAAGU (in which G was [ 32 P]-labelled), nucleotides 2–9 were removed by nuclease P1 digestion, and the caps were separated by thin-layer chromatography (TLC). The controls ( G pppG, G pppG m , m G pppG and m G pppG m , from left to right) were obtained with the same substrate, using MTases that specifically methylate caps at the N 7 or 2′ O positions (human N 7- and vaccinia virus 2′ O -MTase). The TLC experiment used 0.65 M LiCl as mobile phase, allowing a clear separation of m G pppG and m G pppG m (top). The caps on the TLC plate were subsequently further resolved, this time using 0.45 M (NH 2 ) 2 SO 4 as mobile phase for a better separation of G pppG and G pppG m (bottom). G pppG m appears first (after a 1-h incubation), m G pppG m becomes prominent at a later stage, and m G pppG was not observed, indicating that 2′ O -methylation of N 1 precedes N 7-methylation of G . ( b ). The effect of point mutations on the MTase activities of CR-VI+, measured after a 16-h incubation period (by means of a filter-binding assay, as in Fig. 2 ), using G pppGGGACAAGU substrates that were methylated beforehand at N 7 of G or 2′ O of N1, to specifically monitor 2′ O or N 7-MTase activities, respectively. Mutants are listed against a yellow, green or red background, to indicate that the altered residue belongs to λ 1650–1666 , the rest of the CR-VI domain, or the +domain, respectively. They are also grouped according to whether they change the K-D-K-E tetrad, SAM P, SUB P or NS P. The results highlight the importance of essential SUB P residues (such as the K-K-G lysines K 1991 , K 1992 and K 1995 and λ 1650–1666 residues H 1659 and R 1662 ) for both 2′ O - and N 7-methylation. All tetrad residues are crucial for 2′ O -methylation, while D 1779 in particular is important for N7 -MTase activity. The bars and error bars correspond to the mean values from three independent measurements and their s.d.’s, respectively. Full size image Structure of the +domain The crystal structure of CR-VI+ was solved to 2.2 Å resolution in space group P2 1 2 1 2 1 with two molecules, disulphide-linked at residue C 1877 , in the asymmetric unit, assuming a ‘head-to-toe’ conformation ( Supplementary Fig. 1 ). There are no significant differences between the molecules, which have a slightly twisted, bi-lobed shape, composed of two globular domains, the larger corresponding to CR-VI (residues ∼ 1,616–1,883) and the smaller to the +domain (1,884–2,005; Fig. 1b ). Although composed of only ∼ 120 residues in Pneumovirinae , the size of the +domain varies greatly within the Mononegavirales order, reaching ∼ 240 residues in Rhabdoviridae . In hMPV, it consists of six α-helices (α + 1–6). Helix α + 6 contains the K-K-G motif ( Supplementary Fig. 2 ) and together with α + 1 leans over the active cleft of CR-VI. Helix α + 4, and to a lesser extent helices α + 1, α + 5 and α + 6, packs down on λ 1650–1666 , the second half of a long loop (residues 1,635–1,666) that swerves around the CR-VI domain ( Fig. 1b and Supplementary Fig. 3 ; ‘λ’ is used throughout the paper to denote loops). The λ 1650–1666 region, which contains a small helix (α-a), acts as a fulcrum allowing the +domain to pivot relative to the CR-VI domain. Helix α + 3 varies in length, from 4½ turns (in most crystals) to 6 (in Protein Data Bank (PDB) 4UCY), and the loop between α + 2 and α + 3 is always disordered ( Supplementary Fig. 3 ). In crystals of the monomeric C 1877 A mutant (space group P3 1 21), this disordered, unstable region is further enlarged, as helix α + 2 completely unfolds and α + 3 unwinds to 3½ turns. Structure of the CR-VI domain The CR-VI domain shares some peripheral characteristics with the 2′ O -MTases of SARS coronavirus (PDB: 2XYQ) [10] , vaccinia virus (1VP3) (ref. 11 ) and bluetongue virus (VP4-subunit; 2JHA) [12] , such as the long N-terminal loop and the position of helix αX. In its active core, however, it better resembles RrmJ-type flavivirus MTases (for example, 3EVF [9] ; Supplementary Fig. 4 ). Most notably, hMPV and flaviviruses share an unusually long ( ∼ 10 residues), flexible β2 λ (that is, the loop immediately following the β2-strand), which forms the SAM-binding pocket ( SAM P) along with loops β1 λ and β4 λ, shielding it from the solvent ( Fig. 1b, c ). In Wesselsbron (flavi-)virus, β2 λ is found in closed or open conformations, either packing up against SAM (PDB: 3ELW) or exposing it to the solvent (3EMB) [13] , changes that may assist SAM uptake and/or SAH expulsion. In CR-VI+, β2 λ similarly assumes alternate conformations ( Fig. 4c,d ). In the ‘closed’ form, the ligand’s ribose group is hydrogen bonded to D 1725 , and—via a water—to D 1722. Loops β1 λ and β4 λ also show a degree of flexibility. β1 λ residue E 1697 , conserved in paramyxo- and filoviruses, forms a hydrogen bond with the NH 2 group of SAM and is essential for both MTase activities ( Fig. 3b ). However, in the absence of SAM, its side chain either moves into the sub-pocket that normally accommodates the NH 2 group, or, more markedly, turns towards the solvent in the direction of β2 λ, which in this case assumes the ‘open’ position ( Fig. 4d ). β4 λ forms a side wall of SAM P, and together with αD and β5 also defines a deep, hydrophobic cavity not present in other MTases, termed NS P (or nucleoside-binding pocket). Although a role for NS P has yet to be determined, the pocket binds the adenosine moiety of SAM or ATP, soaked at high (25 mM) concentrations into CR-VI+ crystals, causing β4 λ to impinge onto SAM P ( Fig. 4c,d ; when SAM is used for soaking, one SAM molecule occupies SAM P, and another binds to NS P). GTP was not observed in NS P, but this may reflect a lower soaking concentration (2.5 mM), due to GTP’s poor solubility. With the exception of E 1781 , the amino acids lining NS P are poorly conserved beyond the Pneumovirinae , and mutating key NS P residues barely affects the MTase activities ( Fig. 3b ). CR-VI, finally, contains a Zn-finger, which is not conserved beyond the Pneumovirinae subfamily and links the small α–d′ to the rest of the structure ( Fig. 1b ). 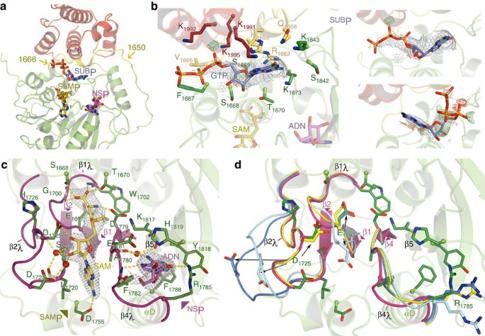Figure 4: CR-VI+-binding pockets. The cartoon representations show the +domain in red and CR-VI in green, with λ1650–1666in yellow. SAM (inSAMP), GTP (inSUBP) and adenosine (ADN; inNSP) are shown as sticks, with the C atoms coloured gold, slate and magenta, respectively. Hydrogens (in white) accentuate the methyl group of SAM. 2Fo-Fc electron density maps around the ligands are represented in grey mesh (contoured at 1σ). (a) The relative positions of the pockets in the protein. (b) Close-up ofSUBP, which is defined by residues of the +domain (particularly the K-K-G motif), λ1650–1666and the CR-VI domain. Residues involved in ligand binding are shown as sticks. GTP is fitted in different orientations into the density in the PDB 4UCZ structure (main figure, and top figure to the right, where the guanosine ring is turned 180°) and in the PDB 4UCI structure (bottom right, where the ligand lays in the opposite direction), highlighting that the ligand can bind in different orientations within the spacious pocket. (c)SAMP andNSP containing a SAM and ADN ligand, respectively (PDB 4UCI, in whichSUBP is also occupied). Residues lining the pockets are shown as sticks. The loops delineatingSAMP (β1λ,β2λ andβ4λ) and the β-strands they originate from are shown in magenta. The dashed yellow lines show putative hydrogen bonds. (d). Superposition of three other CR-VI+ structures onto that inc, highlighting the flexibility ofβ1λ (especially E1697),β2λ andβ4λ. The structure in blue (PDB 4UCK) contains SAM, whereas those in yellow (4UCL) and aquamarine (4UCJ) have emptySAMPs (this suggests that there is no strict correlation betweenSAMP occupancy and the position ofβ2λ).NSP is empty in the three superposed structures, which apparently affects the position of theirβ4λ loops and especially of the R1785side group, which closes the pocket when occupied. All overlaid structures have emptySUBPs. Figure 4: CR-VI+-binding pockets. The cartoon representations show the +domain in red and CR-VI in green, with λ 1650–1666 in yellow. SAM (in SAM P), GTP (in SUB P) and adenosine (ADN; in NS P) are shown as sticks, with the C atoms coloured gold, slate and magenta, respectively. Hydrogens (in white) accentuate the methyl group of SAM. 2Fo-Fc electron density maps around the ligands are represented in grey mesh (contoured at 1σ). ( a ) The relative positions of the pockets in the protein. ( b ) Close-up of SUB P, which is defined by residues of the +domain (particularly the K-K-G motif), λ 1650–1666 and the CR-VI domain. Residues involved in ligand binding are shown as sticks. GTP is fitted in different orientations into the density in the PDB 4UCZ structure (main figure, and top figure to the right, where the guanosine ring is turned 180°) and in the PDB 4UCI structure (bottom right, where the ligand lays in the opposite direction), highlighting that the ligand can bind in different orientations within the spacious pocket. ( c ) SAM P and NS P containing a SAM and ADN ligand, respectively (PDB 4UCI, in which SUB P is also occupied). Residues lining the pockets are shown as sticks. The loops delineating SAM P ( β1 λ, β2 λ and β4 λ) and the β-strands they originate from are shown in magenta. The dashed yellow lines show putative hydrogen bonds. ( d ). Superposition of three other CR-VI+ structures onto that in c , highlighting the flexibility of β1 λ (especially E 1697 ), β2 λ and β4 λ. The structure in blue (PDB 4UCK) contains SAM, whereas those in yellow (4UCL) and aquamarine (4UCJ) have empty SAM Ps (this suggests that there is no strict correlation between SAM P occupancy and the position of β2 λ). NS P is empty in the three superposed structures, which apparently affects the position of their β4 λ loops and especially of the R 1785 side group, which closes the pocket when occupied. All overlaid structures have empty SUB Ps. Full size image During the preparation of this manuscript, a 3.8-Å structure of VSV L , obtained by electron cryo-microscopy, was published [14] . The CR-VI (or MTase) part of VSV resembles that of hMPV, but apparently lacks a deep NS P pocket (PDB: 5a22, Fig. 5 ). The +domain (C-terminal domain) is more elaborate in VSV than in hMPV, containing extra regions N and C terminal of helix α + 6. The helix itself, however, appears well conserved, both in length and in position. Although a K-K-G motif is not present in VSV, it does contain an arginine (R 2038 ) strictly conserved among the Rhabdoviridae , which is structurally equivalent to hMPV’s K 1995 , the second lysine of K-K-G motif. 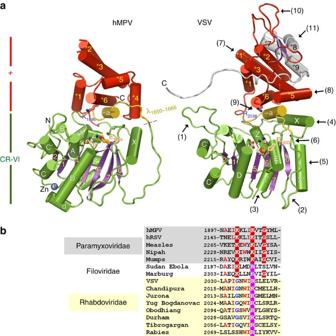Figure 5: Comparison of the CR-VI+ domains of hMPV and VSV. (a). Cartoon representations. The CR-VI domains are similar, and share the unusual, strand-0 containing β-sheet (purple), the rather largeβ2λ—indicated by arrow (1)—and the long N-terminal loop (2), which runs somewhat differently in VSV. The λ1650–1666peptide on which the +domain rests (yellow) also has a homologue in VSV. The Zn-finger, however, is not conserved, and α-helices B and Z are not fragmented. Helix αE, an element of the standard MTase topology (Fig. 1c), is present in VSV (3), as a result of whichNSP may have disappeared. αX is at a different location (4), and is preceded by an extra helix (αx′(5)). E1833, expected to belong to the K-D-K-E tetrad from sequence alignments, is buried in the structure and does not reach the surface of the catalytic pocket (6), and the position normally taken by the K-D-K-E glutamate is occupied by T1831. The +domain of VSV is tilted, compared with that of hMPV, and more elaborate. Helices α+1, α+2, α+3, α+5 and α+6 are conserved, but the α+1–α+2 loop is replaced by an extra helix (α+1′ (7)). α+4 is absent, whereas α+5 is enlarged and immediately follows α+3 (8). The 2-residue loop connecting α+5 and α+6 in hMPV is replaced by a 34-residue coil carrying a small three-stranded β-sheet (9). Helix α+6 seems best conserved between the two +domains, although a K-K-G motif is not present in VSV. However, R2038, which is strictly conserved inRhabdoviridae, takes the place of K1995((10) and alignment below). In VSV, the +domain is extended beyond α+6 with a 65-residue, partly helical, but mainly unstructured polypeptide (in grey (11)). Colour scheme and labelling are as inFig. 1b. (b). Alignment of α+6-helices from MononegaviralesLproteins. K-K-G motif residues are highlighted in red; the arginine replacing the second lysine of the motif inFiloviridaeandRhabdoviridaeis highlighted in magenta. Red letters indicate other (less strictly) conserved residues, except for the G that replaces the first lysine of the K-K-G motif in mostRhabdoviridae(blue). Figure 5: Comparison of the CR-VI+ domains of hMPV and VSV. ( a ). Cartoon representations. The CR-VI domains are similar, and share the unusual, strand-0 containing β-sheet (purple), the rather large β2 λ—indicated by arrow ( 1 )—and the long N-terminal loop ( 2 ), which runs somewhat differently in VSV. The λ 1650–1666 peptide on which the +domain rests (yellow) also has a homologue in VSV. The Zn-finger, however, is not conserved, and α-helices B and Z are not fragmented. Helix αE, an element of the standard MTase topology ( Fig. 1c ), is present in VSV ( 3 ), as a result of which NS P may have disappeared. αX is at a different location ( 4 ), and is preceded by an extra helix (αx′( 5 )). E 1833 , expected to belong to the K-D-K-E tetrad from sequence alignments, is buried in the structure and does not reach the surface of the catalytic pocket ( 6 ), and the position normally taken by the K-D-K-E glutamate is occupied by T 1831 . The +domain of VSV is tilted, compared with that of hMPV, and more elaborate. Helices α + 1, α + 2, α + 3, α + 5 and α + 6 are conserved, but the α + 1–α + 2 loop is replaced by an extra helix (α + 1′ ( 7 )). α + 4 is absent, whereas α + 5 is enlarged and immediately follows α + 3 ( 8 ). The 2-residue loop connecting α + 5 and α + 6 in hMPV is replaced by a 34-residue coil carrying a small three-stranded β-sheet ( 9 ). Helix α + 6 seems best conserved between the two +domains, although a K-K-G motif is not present in VSV. However, R 2038 , which is strictly conserved in Rhabdoviridae , takes the place of K 1995 (( 10 ) and alignment below). In VSV, the +domain is extended beyond α + 6 with a 65-residue, partly helical, but mainly unstructured polypeptide (in grey ( 11 )). Colour scheme and labelling are as in Fig. 1b . ( b ). Alignment of α + 6-helices from Mononegavirales L proteins. K-K-G motif residues are highlighted in red; the arginine replacing the second lysine of the motif in Filoviridae and Rhabdoviridae is highlighted in magenta. Red letters indicate other (less strictly) conserved residues, except for the G that replaces the first lysine of the K-K-G motif in most Rhabdoviridae (blue). Full size image The absence of a classical cap-binding site A common feature of MTases involved in cap methylation is a defined cap-binding pocket that binds G with high affinity, enabling subsequent, low-affinity interactions with the triphosphate bridge and the first few nucleotides, thus precluding methylation of uncapped RNAs [15] , [16] . In CR-VI+, however, an open, solvent-exposed area is found where this pocket is normally located ( Fig. 6a ). Moreover, G pppG- or m G pppG binding was not observed in co-crystallization or soaking experiments, suggesting that CR-VI+ has a weak affinity for G at best and that the cap is not required for substrate recognition. This is consistent with CR-VI+ binding capped and uncapped RNAs with similar strength and being able to 2′ O -methylate uncapped RNAs ( Fig. 2b ). Strong binding would also prevent translocation of G into SUB P for N 7-methylation. Although a high-affinity cap-binding site is clearly absent from CR-VI+, the low-affinity nucleoside binding to NS P and the convenient location of this pocket relative to SUB P suggest it could provide space for G without forming strong interactions ( Supplementary Fig. 5 ). 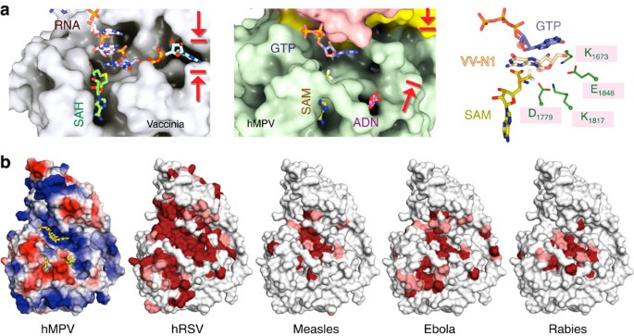Figure 6: RNA-binding site comparisons. (a). Comparison of the RNA-binding sites in vaccinia virus cap-MTase (PDB 1AV6) and CR-VI+. The vaccinia virus MTase (white surface, left) has a narrow cap-binding pocket (in between the red arrows) and a large, open RNA-binding site (adjoining the SAH-containingSAMP). In CR-VI+ (coloured surface, middle) the cap-binding pocket is not present, whereas the RNA-binding site is narrowed (intoSUBP) by the +domain overhang (in red). A structural superposition (obtained by aligning the K-D-K-E tetrads, right) shows that the GTP ligand in CR-VI+ is situated at a considerably greater distance from the tetrad than the first transcribed nucleotide (N1) in the vaccinia virus MTase–RNA complex (shown in light pink). The 2′Oatoms of the nucleotides are shown as transparent, red spheres. (b).SUBP conservation within the Mononegavirales order. The surface presentation on the left shows the basic (blue) and acidic (red) charge distribution on CR-VI+. The ligands are in yellow. The other cartoons show the surface of the hMPV CR-VI+ domain in the same orientation, but in white. Residues that are conserved in the hRSV, Measles, Ebola or Rabies virus homologues of CR-VI+ are coloured dark red (identical residues) or pink (similar residues), and cluster aroundSUBP andSAMP. Figure 6: RNA-binding site comparisons. ( a ). Comparison of the RNA-binding sites in vaccinia virus cap-MTase (PDB 1AV6) and CR-VI+. The vaccinia virus MTase (white surface, left) has a narrow cap-binding pocket (in between the red arrows) and a large, open RNA-binding site (adjoining the SAH-containing SAM P). In CR-VI+ (coloured surface, middle) the cap-binding pocket is not present, whereas the RNA-binding site is narrowed (into SUB P) by the +domain overhang (in red). A structural superposition (obtained by aligning the K-D-K-E tetrads, right) shows that the GTP ligand in CR-VI+ is situated at a considerably greater distance from the tetrad than the first transcribed nucleotide (N 1 ) in the vaccinia virus MTase–RNA complex (shown in light pink). The 2′ O atoms of the nucleotides are shown as transparent, red spheres. ( b ). SUB P conservation within the Mononegavirales order. The surface presentation on the left shows the basic (blue) and acidic (red) charge distribution on CR-VI+. The ligands are in yellow. The other cartoons show the surface of the hMPV CR-VI+ domain in the same orientation, but in white. Residues that are conserved in the hRSV, Measles, Ebola or Rabies virus homologues of CR-VI+ are coloured dark red (identical residues) or pink (similar residues), and cluster around SUB P and SAM P. Full size image The absence of a high-affinity cap-binding pocket appears partly compensated for by the narrowing of the groove that in related MTases accommodates the first few nucleotides of the transcripts, by the overhanging +domain ( Figs 4 and 6a ). In particular, the site adjoining SAM P, which holds the nucleotides undergoing methylation, has become a more elaborate, but narrower and possibly therefore, higher-affinity substrate-binding pocket (termed SUB P as it accommodates the nucleotide undergoing methylation). Consistently, electron density is found in SUB P following soaking or co-crystallization with GTP, whereas in other MTases added GTP predominantly shows up in the cap-binding pocket. In particular, helix α + 6 and the +domain-affiliated λ 1650–1666 help shape SUB P through the side chains of K 1991 and K 1995 (of the K-K-G motif), and of H 1659 and R 1662 , respectively ( Fig. 4b ). The marked decrease in MTase activity of mutants altered at these residues ( Fig. 3b ) illustrates the importance of SUB P in correctly presenting the substrate nucleotides to SAM. Nevertheless, the pocket is too spacious for a single nucleotide, and the electron density in SUB P from a number of soaked crystals suggests that bound GTP often assumes more than one orientation. In structures where GTP could be fitted with confidence, the guanosine moiety predominantly interacts with λ 1650–1666 residues H 1659 and R 1662 , and with K 1991 and (K-D-K-E residue) K 1673 , which clamp the guanine ( Fig. 4b ). Unusually for cap-MTases, K 1673 is not part of αZ, but instead resides on the small z′ (3 10 )-helix ( Fig. 1b,c ). Whether any of the observed positions of GTP reflects in vivo binding of N 1 (as part of a transcript) is unclear; in MTase–RNA complexes (PDB: 1AV6 (ref. 17 ), 4N49 (ref. 16 )), N 1 is situated much closer to the K-D-K-E tetrad ( Fig. 6a ). A potential role of CR-VI+ in cap addition K-K-G residue K 1995 corresponds to the G p binding lysine in the signature motif of eukaryotic GTases, but here is in a loop instead of an α-helix (PDB: 3S24 (ref. 18 ), 1CKN (ref. 19 )) and appears ideally placed to target the phosphate tail of GTP. Although incubation of CR-VI+ with [α- 32 P]- and [β- 32 P]-GTP, in the absence of Mg ++ , resulted in radioactive protein bands on denaturing SDS gels, the level of radioactivity was low, and was not diminished by acid treatment before SDS–polyacrylamide gel electrophoresis (SDS–PAGE), implying it is not due to phosphoamide bond formation. A second, strong argument against a GTase-based capping mechanism in hMPV (and in favour of a PRNTase-based one) is the fact that in the closely related RSV the cap is formed by G pp ligation to pRNA [20] . We observed that CR-VI+ also displays NTPase activity, converting GTP into GDP and ATP into ADP ( Fig. 7 ). GTPase activity, which is required for PRNTase-based capping, was previously reported in Mononegavirales L (ref. 21 ), but as yet could not be linked to a specific domain within the protein. The reaction observed with CR-VI+, however, is quite slow, possibly because other parts of L , or other co-factors, are needed for full activity. In line with this, we were not able to identify key active-site residues. Using the mutants listed in Fig. 3b , the greatest reductions in GTPase activity were obtained with E 1697 C (corresponding to the flexible residue at the bottom of SAM P; Fig. 4d ) and S 1669 A (part of SUB P, Fig. 4b ) to 54 (±20) and 57 (±16) % of the wild-type activity, respectively ( n =3). The deletion of the dipeptide G 1645 K 1646 from the long N-terminal loop resulted in a somewhat more pronounced ∼ 70% reduction ( Supplementary Fig. 6 ). The NTPase activity was confirmed using crystallized CR-VI+ ( Fig. 7 ). 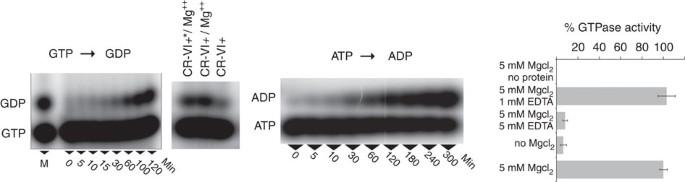Figure 7: NTPase activity. Autoradiographs of urea–PAGE gels show CR-VI+-mediated conversion of radiolabelled GTP to GDP and ATP to ADP, over time. The smaller autoradiograph shows the requirement of Mg++for the reaction (allowed to proceed for 1 h), and also shows efficient GDP generation by washed, dissolved CR-VI+ crystals (CR-VI+*), dispelling the possibility that the activity is due to contaminants. The diagram on the right (obtained by phosphorimage analysis following electrophoresis) further illustrates the requirement of Mg++and shows the effect of the metal-ion chelator EDTA on the GTPase reaction. The bars and error bars correspond to the mean values from three independent measurements and their s.d.’s, respectively. Figure 7: NTPase activity. Autoradiographs of urea–PAGE gels show CR-VI+-mediated conversion of radiolabelled GTP to GDP and ATP to ADP, over time. The smaller autoradiograph shows the requirement of Mg ++ for the reaction (allowed to proceed for 1 h), and also shows efficient GDP generation by washed, dissolved CR-VI+ crystals (CR-VI+*), dispelling the possibility that the activity is due to contaminants. The diagram on the right (obtained by phosphorimage analysis following electrophoresis) further illustrates the requirement of Mg ++ and shows the effect of the metal-ion chelator EDTA on the GTPase reaction. The bars and error bars correspond to the mean values from three independent measurements and their s.d.’s, respectively. Full size image As a GDP is transferred onto a PRNTase-bound pRNA intermediate during cap synthesis in VSV [21] , the presence of NTPase activity in CR-VI+ would suggest that this domain is involved in cap addition. It is unclear from the structure of VSV L how capping, cap methylation and RNA synthesis are coordinated [14] , but an involvement of CR-VI+ in cap addition is consistent with the dynamic nature of the multi-domain polymerases of RNA viruses in general, exemplified by flu where the C-terminal two-thirds of PB2 has been shown to be extremely mobile [22] , [23] . The presentation of uncapped (but CR-V-linked) pRNA to CR-VI+ would also explain why hMPV L does not require a high-affinity cap-binding site. The integrity of both the PRNTase and K-K-G motifs, moreover, has been shown to be essential for viable mRNA synthesis in human parainfluenzavirus 2 (hPIV-2) 5 , in line with capping involving a concerted action of CR-V and CR-VI+. Assuming the transcript is presented to CR-VI+ by the PRNTase, 2′ O -methylation may actually occur before the cap is added (as a cap is not required for the reaction; Fig. 2b ), which would also be consistent with 2′ O -methylation preceding N 7-methylation. The possibility that 2′ O -methylation precedes cap addition was also suggested by the ability of virions of the rhabdovirus spring viremia of carp virus to synthesize uncapped, N1-methylated oligonucleotides [24] . We did not observe significant methylation of free GTP by CR-VI+ (levels were <5% of that of G pppGGGACAAGU methylation), suggesting G N 7-methylation takes place after G is added to the RNA. In addition 2′ O -methylated substrates ( G pppG m GGACAAGU and pppG m GGACAAGU) show an ∼ 2-fold higher affinity for CR-VI+, compared with their unmethylated counterparts ( Fig. 2b ), which presumably reflects an RNA repositioning mechanism allowing the G N 7 atom access to the SAM methyl donor in the second methylation step. In conclusion, CR-VI+ is a dynamic part of the L protein that potentially completes PRNTase-initiated cap addition, and methylates the cap at its 2′ O and N 7 positions. The SUB P pocket, which is conserved among Paramyxoviridae and Filoviridae ( Fig. 6b ), is clearly instrumental in key activities of the domain, and thus represents an attractive target for the structure-based design of (potentially broad-spectrum) antiviral compounds. Cloning and expression The sequence encoding CR-VI+ was PCR amplified using primers that added a C-terminal SGHHHHHH-tag to the translation product, from a synthetic hMPV L gene ( hMPV isolate 00-1 , GenBank: AF371337.2), codon optimized for expression in Spodoptera frugiperda ( Sf ) cells (Geneart). The amplicon was cloned into pOPIN-E for expression in HEK293T mammalian cells (following transfection using Lipofectamine 2000; Invitrogen), in BL21 Star bacteria (Invitrogen) and in Sf 21 (insect cells) following co-transfection with (flashBACULTRA) baculovirus (Oxford Expression Systems) using Cellfectin II (Invitrogen) [25] . Mutants were generated by PCR, using primers carrying the mutation ( Supplementary Fig. 7 ). The CR-VI+ DNA was used as a template for mutagenesis, except for the K 1991 Q/K 1995 Q and K 1991 Q/K 1992 Q/K 1995 Q mutants, which were obtained using the K 1995 Q DNA. For each mutation, the forward primer was combined with a vector-specific reverse primer (5′-AGTGGTATTTGTGAGCCAGG-3′), and, in a second PCR, the reverse primer was used together with a vector-specific forward primer (5′-CCTTTAATTCAACCCAACAC-3′). The two PCR products thus generated were digested with either BspQI or BtsI (New England Biolabs), restriction enzymes that cut within the CR-VI+-specific primer regions. The amplicons were then rejoined using T4 DNA ligase (New England Biolabs), and the ligation products were PCR amplified using the vector-specific primers for insertion in the pOPIN-E vector. Purification Seventy-two hours after infection of the suspension cultures with recombinant baculovirus, Sf 21 cells were spun down (1,000 g , 7 min, 22 °C) and lysed in one-fourth volume of buffer L (1.5% triton X-100, 5% glycerol, 50 mM arginine, 300 mM KCl, 10 mM imidazole and 20 mM Tris (pH 8.0)). After clarification (10,000 g , 25 min, 4 °C), the lysate was incubated with benzonase (Novagen; to 0.2 U ml −1 ) and NiNTA resin (Qiagen; 0.3 ml l −1 culture) for 5 h at 4 °C, with gentle shaking. The beads were transferred to a 10-ml column and washed with 3 × 10 ml buffer W (20 mM Tris (pH 8.0), 1.5 M NaCl, 10 mM imidazole and 7.5% glycerol) and 1.5 ml of 0.1 M arginine (pH 8.0). Protein was eluted in 0.8 M arginine (pH 8.0). An equal volume of ice-cold 3 M AmSO 4 was added to the eluent, and the precipitated protein collected (10,000 g , 10 min, 4 °C). Protein pellets were stored at −20 °C. A similar lysis and purification protocol was used to obtain recombinant protein from HEK293T cells. BL21 Star cells were lysed using Bugbuster Protein Extraction Reagent (Novagen). Expression and purification were monitored by SDS–PAGE and western blotting. Blots were developed with a 1/10,000 dilution of an anti-histidine tag antibody (Penta·His Antibody, Qiagen, catalogue number 34660). Supplementary Fig. 1 shows purified protein following SDS–PAGE under reducing and non-reducing conditions. An uncropped western blot showing the unreduced, insect-cell-expressed protein next to a BenchMark (Invitrogen) molecular weight marker is also shown. Selenomethionine incorporation Twenty hours following infection of an Sf 21 suspension culture (27.8 °C, with an agitation speed of 130 r.p.m./0.25 g ), cells were collected (70 g , 10 min, 22 °C) and resuspended in cysteine- and methionine-free SF900II medium (Gibco) supplemented with dialysed fetal bovine serum (Gibco; 7% v/v) and 150 mg l −1 L -cysteine (Sigma). Following an additional 4 h at 27.8 °C in the shaking incubator, 250 mg l −1 selenomethionine (Sigma) was added. Protein expression was allowed to continue for another 48 h. Proteins were purified as above. Crystallization, structure solving, refinement and validation Crystallization was carried out by vapour diffusion at 20.5 °C using 96-well sitting drop plates (Greiner) [26] . Protein pellets were dissolved in water to 5–6 mg ml −1 , and initial crystals were obtained by equilibrating 100 nl of protein with 100 nl of reservoir solution C11 of the PGA-HT screen (Molecular Dimensions; pH 6.5) supplemented with guanidine hydrochloride (to 0.1 M), against 0.1 ml of reservoir. Glycerol was added (to 20% v/v) for cryoprotection. Diffraction data were collected at 100 K on Diamond beamlines I02, I03, I04 and I24 (Harwell, UK), and processed using the Xia2 programme suite [27] . A single-wavelength anomalous dispersion experiment allowed determination and refinement of the positions of selenium atoms, as well as calculation of the phases with autoSHARP [28] . An initial model was obtained using MR-ROSETTA [29] , enabling manual model building using COOT [30] . Refinement was performed using autoBUSTER [31] , and validation employed COOT and Molprobity [32] . Molecular replacement (using PHASER [33] ) was used to solve additional CR-VI+ structures. Refinement statistics are given in Table 1 , and a portion of the electron density map is shown in Supplementary Fig. 8 . Table 1 Crystallographic data collection and refinement statistics. Full size table Synthesis of RNA substrates RNA sequences were chemically synthesized on a solid support using an ABI 394 synthesizer. After RNA elongation with 2′ O -pivaloyloxymethyl phosphoramidite monomers [34] , [35] (Chemgenes, USA), the 5′-hydroxyl group was phosphorylated and the resulting H -phosphonate derivative [36] oxidized and activated into a phosphoroimidazolidate derivative to react with either phosphoric acid (for ppRNA synthesis), pyrophosphate (pppRNA) [36] or guanosine diphosphate ( G pppRNA) [37] , [38] . N 7-methylation of the purified G pppRNA was performed enzymatically using N 7-hMTase [37] , [38] . To prepare monophosphate RNA (pRNA), the 5′- H -phosphonate RNA was treated with a mixture of N , O -bis-trimethylacetamide (0.4 ml), CH 3 CN (0.8 ml) and triethylamine (0.1 ml) at 35 °C for 15 min, and then oxidized with a tert -butyl hydroperoxide solution (5–6 M in decane, 0.4 ml; 35 °C, 15 min). After deprotection and release from the solid support, RNA sequences were purified by IEX-HPLC (>95% pure) and their identity were confirmed by MALDI-TOF (Matrix-Assisted Laser Desorption/Ionization Time-of-Fight) spectrometry. MTase activity assays These were performed by combining 4 μM CR-VI+ with 0.7 μM of the purified and validated synthetic RNAs, 10 μM SAM and 0.33 μM 3 H-SAM (Perkin Elmer) in 40 mM Tris-HCl (pH 8.5) and 1 mM dithiothreitol (DTT). Reactions (at 30 °C) were stopped by a 10-fold dilution in 100 μM ice-cold SAH and the samples were transferred to DEAE filtermats (Perkin Elmer) using a Filtermat Harvester (Packard Instruments). The RNA-retaining mats were washed twice with 10 mM ammonium formate (pH 8.0), twice with water and once with ethanol. They were then soaked with liquid scintillation fluid, allowing the measurement of 3 H-methyl transfer to the RNA substrates using a Wallac MicroBeta TriLux Liquid Scintillation Counter [13] . Methylation of GTP was determined in the same buffer (minus the 3 H-SAM and RNA), using the EPIgeneous methyltransferase assay kit (Cisbio), which measures the generation of SAH, as it competes with d2-coupled SAH for binding to a Lumi4-Tb-labelled anti-SAH antibody, affecting the TR-FRET signal between these compounds. In practice, MTase reactions were stopped after 16 h by addition of the detection reagents, and 1 h later the TR-FRET signal was monitored using a PHERAstar Flashlamp plate reader. Thin-layer chromatography analysis of cap structures G *pppGGGACAAGU (in which the asterisk indicates the [ 32 P]-labelled phosphate) was synthesized by incubating pppGGGACAAGU (10 μM) with vaccinia virus capping enzyme (New England Biolabs) in the presence of 1.65 μCi [α- 32 P]-GTP (Perkin Elmer). The capped RNA was purified by precipitation in 3 M sodium acetate supplemented with 1 μg μl −1 of glycogen (Thermo Scientific), and submitted to methylation by CR-VI+ (as above), after which it was precipitated again (stopping the reactions), and digested with 1 U of Nuclease P1 (US Biologicals) in 30 mM sodium acetate (pH 5.3), 5 mM ZnCl 2 and 50 mM NaCl (4 h, 37 °C). The products were spotted onto polyethylenimine cellulose thin-layer chromatography plates (Macherey Nagel), and resolved in two steps, first using 0.65 M LiCl, then 0.45 M (NH 2 ) 2 SO 4 as mobile phase. The radiolabelled caps released by nuclease P1 were visualized using a Fluorescent Image Analyzer FLA3000 (Fuji) phosphor-imager. Characterization of RNA-CR-VI+ interactions Using T4 RNA ligase 1 (20 units; New England Biolabs), [5′- 32 P]-pCp (1.1 μCi) was ligated to the 3′-ends of the RNA substrates (10 μM) in 50 mM Tris-HCl (pH 7.8), 10 mM MgCl 2 , 10 mM DTT and 1 mM ATP (16 °C, overnight). Ligase was removed by RNA precipitation in 3 M sodium acetate supplemented with 1 μg μl −1 of glycogen (Thermo Scientific). The radiolabelled RNA was incubated (15 min, 37 °C) with increasing concentrations of CR-VI+, in 20 mM Tris-HCl (pH 8.5), 1 mM DTT, 10% glycerol and 30 mM NaCl. The reaction mixtures were spotted onto nitrocellulose (GE Healthcare) using a manifold-1 dot-blot apparatus (Whatman) and washed with 20 mM Tris-HCl (pH 8.5), 1 mM DTT and 50 mM NaCl. Membrane-bound RNA was quantified by phosphor-imaging. Dissociation constants ( K D s) were determined using Hill slope curve fitting (Prism). NTPase assay Samples combining CR-VI+ (4 μM) with 0.5 μCi [α- 32 P]-GTP or 0.5 μCi [α- 32 P]-ATP in 40 mM Tris-HCl (pH 8.5), 1 mM DTT and 5 mM MgCl 2 were incubated at 37 °C. Reactions were stopped by adding an equal volume of formamide/EDTA gel-loading buffer, and hydrolysis products were separated over a 20% polyacrylamide/8 M urea gel before phosphor-imaging. Accession codes: Coordinates and structure factors are deposited in the Protein Data Bank under accession codes 4UCI , 4UCL , 4UCJ , 4UCK , 4UCZ , 4UCY and 4UD0 . How to cite this article: Paesen, G. C. et al . X-ray structure and activities of an essential Mononegavirales L -protein domain. Nat. Commun. 6:8749 doi: 10.1038/ncomms9749 (2015).